Reply to: Pitfalls in using phenanthroline to study the causal relationship between promoter nucleosome acetylation and transcription 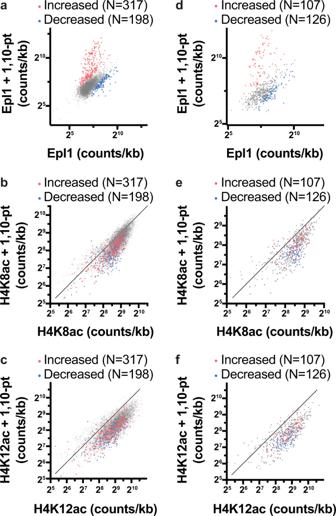Fig. 1: Transcription inhibition by 1,10-phenanthroline (1,10-pt) does not impact Epl1 occupancy at most promoters. Scatter plots comparing the effect of 1,10-pt on fragment midpoint counts from Epl1 (a,d), H4K8ac (b,e), or H4K12ac (c,f) ChIP-seq, over promoters (aandd) or associated +1 nucleosomes (b,c,e, andf) of all (5542) genes (a,b,c) or of 562 genes with NDR Epl1 peaks identified in MNase ChIP-seq in control cells (d,e,f). Promoters with >1.5 fold-change in Epl1 using an adjustedp-value < 0.1 (DESeq2’s binomial test2) are shown in red (increased) or blue (decreased). Inb,c,e, andf, the line is:y=x+ 0. 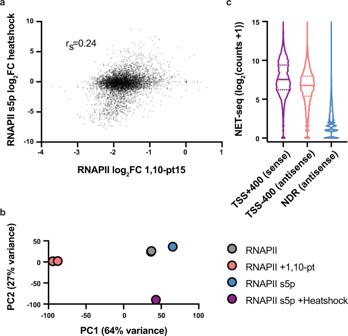Fig. 2: Transcription inhibition with 1,10-phenanthroline (1,10-pt) does not mirror the effect of heat shock on RNAPII occupancy at most genes. aScatter plot comparing the log2fold change (FC) in RNAPII occupancy following treatment with 1,10-pt with RNAPII serine 5 phosphorylation (s5p) following heat shock in gene 5′ regions (TSS to +400 bp) for all (5542) genes.bPCA plot showing the first two principal components calculated across TSS to +400 bp for all (5542) genes.cNET-seq 3′ read counts from TSS to +400 nt (sense), TSS to −400 nt (antisense), or in NDRs (antisense) depicted by violin plots for all (5542) genes. FASTQ files were mapped as described in Martin et al. BAM files were filtered for 100–500 bp reads and total read midpoints overlapping nucleosome depleted regions [4] or +1 nucleosomes [14] , were calculated using the Java Genomics Toolkit ( https://github.com/timpalpant/java-genomics-toolkit ) ngs.IntervalStats script. For DEseq2 analysis [2] , size factors accounting for sequencing depth and the scaling factors reported in Martin et al. [1] were used. For calling NDRs with increased or decreased Epl1 binding, we used lenient cutoffs of a fold change of >1.5 and an adjusted p -value (FDR) of <0.1. For NET-seq data [15] , processed bedGraphs were downloaded from GSM1673641 and GSM1673642. Sense and antisense read counts in specified windows were calculated using the Java Genomics Toolkit, summed across replicates, and violin plots made in Prism. For RNAPII serine 5 phosphorylation ChIP-seq [5] , FASTQ files were downloaded from the SRA (SRR8450263 and SRR8450261) and mapped using BWA. Fragment centers, estimated using an assumed fragment length of 150 bp, were counted from the TSS to +400 bp. These were depth normalized to compare to RNAPII normalized as described in Martin et al. Principal component analysis (PCA) was performed on all 5542 genes (TSS+400) using the regularized log transformation and plotPCA functions of DEseq2 [2] . Reporting summary Further information on research design is available in the Nature Research Reporting Summary linked to this article.